Biosynthesis of DHGA12and its roles inArabidopsisseedling establishment Seed germination and photoautotrophic establishment are controlled by the antagonistic activity of the phytohormones gibberellins (GAs) and abscisic acid (ABA). Here we show that Arabidopsis thaliana GAS2 (Gain of Function in ABA-modulated Seed Germination 2), a protein belonging to the Fe-dependent 2-oxoglutarate dioxygenase superfamily, catalyzes the stereospecific hydration of GA 12 to produce GA 12 16, 17-dihydro-16α-ol (DHGA 12 ). We show that DHGA 12 , a C 20 -GA has an atypical structure compared to known active GAs but can bind to the GA receptor (GID1c). DHGA 12 can promote seed germination, hypocotyl elongation and cotyledon greening. Silencing and over-expression of GAS2 alters the ABA/GA ratio and sensitivity to ABA during seed germination and photoautotrophic establishment. Hence, we propose that GAS2 acts to modulate hormonal balance during early seedling development. Seed germination and subsequent photoautotrophic development of seedlings are complex early developmental processes crucial to subsequent success in the plant life cycle [1] . The antagonistic roles of the phytohormones abscisic acid (ABA) and gibberellins (GAs) in seed germination and seedling development, and their complex regulatory networks, have been the focus of intense research [2] . It is widely accepted that ABA promotes the onset of dormancy and inhibits germination, whereas GA prevents dormancy and stimulates germination [3] , [4] , [5] , [6] . The overall ABA/GA balance in the seed is tightly controlled, since it ultimately dictates its developmental fate, and this balance can be altered by modifying the ratio of endogenous ABA/GA levels, and/or affecting intrinsic sensitivities to either hormone [6] . After germination, seedlings must rapidly develop efficient root systems and establish photoautotrophic capability to adapt to their environment, thereby maximizing their chances of survival [7] . When young seedlings emerge from the ground, they experience dramatic environmental changes that trigger multiple developmental processes, including cotyledon opening, chloroplast development, and leaf de-etiolation. The molecular mechanisms that control the ABA/GA balance in response to environmental factors during the heterotrophic-to-autotrophic transition are mostly unexplored [8] . Existing GAs are derivatives of diterpenoid carboxylic acids, and possess a C3-hydroxyl group [9] . The early steps of biosynthesis, involving ent -copalyl diphosphate synthase (CPS), ent -kaurene synthase (KS) and ent -kaurene oxidase (KO), are each encoded by a single gene in Arabidopsis . Mutants defective in these genes ( ga1 , ga2 , and ga3 ) display severe GA-deficient dwarfing [10] . In contrast to the early GA-biosynthetic enzymes, the GA 20-oxidases (GA20oxs) and GA 3-oxidases (GA3oxs) catalyzing the late steps of the pathway belong to separate gene families within the 2-oxoglutarate-dependent dioxygenases (2ODDs). Their Arabidopsis mutants ( ga4 and ga5 ) develop a semi-dwarf phenotype and can germinate without the addition of exogenous GAs [11] . Considerable progress has been made in the discovery of naturally occurring GA structures, with their numbers now reaching 136, although their physiological functions are mostly unknown [12] . Remarkably, no novel GAs or GA modification routes linked to developmental regulation have been discovered in over 10 years, although it is logical to hypothesize the existence of additional undiscovered natural GAs as well as novel routes to allow their precise regulation. GA20ox proteins have been identified in a large variety of plants [13] . Of the five Arabidopsis GA20oxs, four (GA20ox1, GA20ox2, GA20ox3, and GA20ox4) have GA20ox activity, whereas GA20ox5 has only partial activity [14] , [15] . Expression profiles and mutant analysis indicated functional redundancy of AtGA20ox1 , AtGA20ox2 , and AtGA20ox3 , with all playing key roles in GA biosynthesis and plant development. In contrast, the low expression levels of AtGA20ox4 and AtGA20ox5 explain their less prominent role in development [14] . Although the pathways for the synthesis of bioactive GAs catalyzed by the GA20ox subfamily have been extensively studied [16] , [17] , the roles of more than 100 remaining 2ODD gene family members are still largely unknown [18] . Here, we describe the characterization of “Gain-of-function in ABA-modulated Seed germination 2” ( GAS2 , hereafter) that shows lowered sensitivity to ABA in germination and early seedling development in overexpressing lines than WT, but enhanced ABA sensitivity in loss-of-function mutants of GAS2 . It encodes a Fe-dependent 2-oxoglutarate dioxygenase that catalyzes the biosynthesis of an atypical bioactive GA, named GA 12 16, 17-dihydro-16α-ol (DHGA 12 ). We show that DHGA 12 can bind the GA receptor and to a certain extent promotes seed germination and hypocotyl elongation, as well as enhancing cotyledon greening and seedling development. We propose that GAS2 modulates both the ABA/GA ratio and ABA sensitivity influencing early developmental events in seedlings. Further characterization suggests the possibility that DHGA 12 is involved in the modulation of seedling establishment. GAS2 negatively regulates ABA sensitivity With the aim of finding modulators of ABA signaling, we produced an extensive collection of transgenic Arabidopsis lines carrying the chemically (17-β-estradiol, E2) inducible XVE system [19] adjacent to the T-DNA border. Preliminary experiments established 0.5 µM ABA as the optimal concentration for screening based on its inhibition of seed germination and cotyledon greening (Supplementary Fig. 1a ). Screening of 38,000 T-DNA seeds sown onto Murashige and Skoog (MS) agar plates supplemented with 0.5 µM ABA and 5 µM E2 identified 35 ABA-insensitive plants. One of these showed strong ABA insensitivity during germination and seedling development, and was named Gain of Function in ABA-modulated Seed Germination 2 ( gas2 -D) (Fig. 1a, c ). Homozygous seeds were obtained for the gas2 -D T-DNA line and re-tested under more stringent conditions (1 µM ABA) to confirm the E2-inducible phenotype (Supplementary Fig. 1b ). Seed germination and cotyledon development was strongly inhibited in wild-type (WT) and noninduced gas2 -D plants plated on MS medium supplemented with either 0.2, 0.5 or 1 µM ABA, whereas the addition of E2 blocked the effect of ABA (Fig. 1a–f and Supplementary Figs. 1b , 2a–d ). Growth of wild-type seedlings was arrested by 0.5 µM ABA even when treatment was done following radicle emergence (Fig. 1a, c ). In contrast, treatment with ABA did not significantly delay germination of gas2 -D seeds, nor did it arrest the autotrophic transition and seedling establishment of gas2 -D under E2-inducing conditions (Fig. 1a, c ). No obvious differences in germination and early seedling development were apparent between E2-induced gas2 -D and WT plants grown on MS medium (Fig. 1a, b ). Fig. 1 GAS2 modulates the sensitivity to ABA in seed germination and seedling establishment. a Phenotypes of 10-d-old seedlings of wild-type, E2-induced gas2 -D and two GAS2 overexpression transgenic lines ( GAS2 -OE1 and OE2), grown on MS in absence (Mock) or presence of 0.5 µM ABA (ABA). Bar = 1.5 cm. b , c Cotyledon greening analysis of 10-d-old seedlings of wild-type, E2-induced gas2 -D and two GAS2 overexpression lines ( GAS2 -OE1 and OE2) grown on MS with or without the addition of 0.5 µM ABA. Error bars represent SD (standard deviations) ( n = 72). d Phenotypes of 8-d-old seedlings of wild-type, noninduced gas2 -D, gas2-1 and gas2-2 , grown on MS in absence (Mock) or presence of 0.2 µM ABA (ABA). Bar = 1.5 cm. e Cotyledon greening analysis of 8-d-old seedlings of wild-type, noninduced gas2 -D, gas2-1 and gas2-2 grown on MS in absence (Mock) or presence of 0.2 µM ABA (ABA). Error bars represent SD (standard deviations) ( n = 72). f Seed germination analysis of wild-type, noninduced gas2 -D, gas2-1 and gas2-2 , grown on MS in absence (Mock) or presence of 0.2 µM ABA (ABA) at 48 h. Error bars represent SD (standard deviations) ( n = 72). E2 stands for 17-β-estradiol. * P < 0.05, *** P < 0.001, t test versus mock ( e and f ). Source data are provided as a Source Data file. ABA abscisic acid, MS Murashige and Skoog agar Full size image The position of the T-DNA insertion in the gas2 -D line was determined by thermal asymmetric interlaced polymerase chain reaction (TAIL-PCR), establishing its location in the promoter region of the Arabidopsis gene At2g36690 /GAS2 (Supplementary Fig. 1c–e ) with the trans-activator region localized ~157 bp upstream of the GAS2 start codon (Supplementary Fig. 1c ). GAS2 encodes a member of the 2ODD protein family, showing 45.6% sequence identity to GA20ox1 in the conserved DIOX_N (Non-haem dioxygenase N-terminal domain) and 2OG-FeII_Oxy (Oxoglutarate/iron-dependent dioxygenase) domain (Supplementary Fig. 1g ) [16] , [17] . Expression analysis confirmed that GAS2 transcript levels in gas2- D plants were highly induced by treatment with E2, being 5-6 folds higher than WT (Supplementary Fig. 1f ). Interestingly, the proximity of the T-DNA to the start of transcription resulted in almost complete silencing of GAS2 in the absence of the inducer E2 (Supplementary Fig. 1f ). To confirm that the ABA-insensitive phenotype was due to the overexpression of GAS2 , ten independent transgenic lines were produced by placing the GAS2 cDNA under the control of the cauliflower mosaic virus (CaMV) 35S promoter and two independent lines, GAS2 -OE1 and GAS2 -OE2, with high GAS2 expression levels (Supplementary Fig. 1f ) were selected for further study. The GAS2 -OE lines displayed an ABA-insensitive phenotype similar to that observed for the gain-of-function gas2 -D line in the presence of E2 (Fig. 1a–c ). The noninduced gas2 -D line was treated as a knockdown mutant given the strong downregulation of GAS2 expression caused by the T-DNA insertion (Supplementary Fig. 1c, f ). We produced two more loss-of-function mutants using CRISPR/Cas9 technology ( gas2-1 and gas2-2 , hereafter). Sequencing of T2 homozygous lines identified a 1 bp deletion in gas2-1 and a 1 bp insertion in gas2-2 , leading in each case to frameshifts and complete GAS2 loss-of-function (Supplementary Fig. 1c ). ABA-induced inhibition of cotyledon development and seed germination was more severe in the knockdown ( gas2 -D) plants than WT. As expected, these ABA-induced phenotypes were even more pronounced in the gas2-1 and gas2-2 lines than gas2 -D (Fig. 1d–f and Supplementary Fig. 2a–d ). Overall, our data show that loss-of-function or knockdown mutants of GAS2 are slightly hypersensitive to ABA during germination and early seedling development, whereas the gain-of-function and overexpressing lines are less sensitive to ABA than WT (Fig. 1 and Supplementary Fig. 2 ), suggesting that GAS2 negatively regulates ABA sensitivity during germination, phototrophic establishment and seedling development. GAS2 functions in germination and early seedling development Phenotypic analysis of transgenic Arabidopsis GAS2 knockout and overexpressing lines showed clear alterations in germination and early seedling development. When seeds were allowed to fully dry for several weeks after harvesting, germination of gas2-1 and gas2-2 seeds was slower than WT seeds (29 and 23% vs. 83%, 48 h after stratification in MS) (Fig. 2a ). In contrast, GAS2 -OE1 and GAS2 -OE2 overexpression lines showed faster germination than WT (21 and 15% vs. 0% under the same conditions 36 h after stratification in MS) (Fig. 2a ). Fig. 2 Silencing and overexpression of GAS2 affects seed germination and cotyledon greening. a , b Seed germination and cotyledon greening analysis of wild-type, gas2-1 , gas2-2 and two GAS2 overexpression lines ( GAS2 -OE1 and OE2) grown on MS. Error bars represent SD (standard deviations) ( n = 72). c , d Germination analysis of wild-type, noninduced gas2 -D and overexpressing GAS2 fresh seeds (not allowed to dry) at the 2-d timepoint after sowing with no stratification ( c ) and stratification (at the 3-d timepoint after sowing) ( d ). Error bars represent SD ( n = 108). ** p < 0.01, *** p < 0.001, t test. e Relative GAS2 mRNA levels in roots (R), shoots (Sh), leaves (L), inflorescences (I), siliques (Si) and seeds (Se) analyzed by RT-qPCR. Error bars represent SD. f Relative GAS2 mRNA levels in hypocotyls of Arabidopsis after different light/dark treatment (dark 9 d, dark 9 d + light 6 h, dark 9 d + light 12 h and dark 9 d + light 24 h). The dark 9-d level was arbitrarily adjusted to 1 and the remaining levels were normalized to that value. Error bars represent SD. ** p < 0.01, *** p < 0.001, t test. g Relative GAS2 mRNA levels of the seedlings in response to red and far-red light exposure, analyzed by RT-qPCR. Error bars represent SD. ** p < 0.01, t test. Mock: Far red light 0 h; T1: Far red light 2 h; T2: Far red light 2 h + red light 2 h; T3: Far red light 2 h + red light 2 h + Far red light 2 h. Source data are provided as a Source Data file. MS Murashige and Skoog agar Full size image Similar differences were also evident when fresh seeds (not allowed to dry) were analyzed (Fig. 2c ). In the absence of stratification, gas2 -D seeds, with strong GAS2 downregulation, showed a 50% reduction in germination compared with WT 48 h after sowing, whereas the germination rates of GAS2 -OE1 and GAS2 -OE2 lines were twice that of the WT (Fig. 2c ). All lines achieved 100% germination 3 days after stratification (Fig. 2d ). Early seedling development, measured as the percentage of cotyledon greening, was also altered in the transgenic lines with GAS2 -OE1 and GAS2 -OE2 overexpressing lines showing 69 and 62% values 3 days after germination, as compared with 3% for WT seedlings; the mutant gas2-1 and gas2-2 lines showed a delay in cotyledon greening (Fig. 2b ). As mentioned above, GA 20-oxidases belong to a large class of Fe-containing enzymes, found in plants and fungi, that share a common mechanism of action [18] . Bioinformatics analysis revealed that GAS2 is a member of the 2OG-Fe-dependent oxygenase family, distantly related to GA20oxs (Supplementary Fig. 3 ). Five GA20ox enzymes have been characterized in Arabidopsis , and three of them play important roles in the regulation of active GA levels, having profound effects on vegetative development [14] . Phylogenetic analysis reveals that GAS2 belongs to a subfamily (designated as the GAS2 subfamily) different to that of the GA 20-oxidases. To assess GAS2 expression, we performed reverse transcription quantitative polymerase chain reaction (RT-qPCR) analysis using samples taken from different Arabidopsis tissues. Very low levels of GAS2 expression were detected in all tissues, with the exception of roots and leaves (Fig. 2e ). These results are consistent with Arabidopsis microarray data archived in the BAR eFP browser ( http://bar.utoronto.ca/efp/cgi-bin/efpWeb.cgi ) (Supplementary Fig. 4a, b ) [20] . Previous microarray expression studies indicate that light induces the expression of GAS2 under long day conditions (Supplementary Fig. 4c ). Plants kept in darkness for 9 days displayed an initial reduction in GAS2 transcript levels 6 h after light exposure, followed by a dramatic increase after 12 h of continuous light with high levels maintained after 24 h (Fig. 2f ). It is well established that Arabidopsis germination is inhibited by far-red light and promoted by red light [21] , [22] consistent with our results showing that GAS2 expression was repressed by far-red light whereas treatment with red light reversed the effect, inducing expression two folds over normal levels (Fig. 2g ). Characterization of transgenic Arabidopsis lines carrying 3.96 kb of the GAS2 genomic region, including the promoter and gene sequences fused to the β-glucuronidase (GUS) reporter gene (Supplementary Fig. 5a–c ) showed induction of GUS staining by ABA whereas GA 4 treatment almost completely abolished it (Supplementary Fig. 5a–c ). GAS2 catalyzes the hydration of GA 12 To investigate whether GAS2 exhibits enzymatic activity in GA biosynthesis, we designed several in vitro and in vivo experiments. In a first set of experiments, we performed in vitro biosynthetic assays using the purified GAS2 protein, cofactors, and three different deuterium-labeled substrates. Reaction mixtures containing GA 12 as substrate were collected 0, 5, 30 and 120 min after the start of the reaction. Liquid chromatography-mass spectrometry (LC-MS) analysis showed the gradual appearance of a newly formed peak with a retention time of 70.56 min (Fig. 3a–d ), and a progressive decline in GA 12 levels (Fig. 3e ). Negative control reactions using either denatured GAS2, lacking cofactors, or containing EDTA as an Fe chelator failed to yield any products (Supplementary Fig. 6a–e ). No catalytic products were detected in the reactions containing GA 15 or GA 24 as substrates when analyzed by LC-MS (Supplementary Fig. 7a–h ). To investigate whether GA 12 can act as an endogenous substrate for GAS2, we transiently expressed a GAS2-GFP fusion ( 35 S::GAS2-GFP ) in WT Arabidopsis protoplasts in medium containing GA 12 . MALDI FTICR-MS analysis revealed the appearance of a peak with of m/z 349.201, obtained from full-scan MS (Fig. 3f ), identical to the synthetic GA 12 derivative standard (Supplementary Fig. 8 ). Transient expression of 35 S::GFP in the presence of GA 12 produced a small amount of the GA 12 derivative, perhaps due to enzymatic conversion of GA 12 by endogenous GAS2 (Fig. 3i ). When protoplasts from the GAS2 -OE1 overexpressing line were incubated with GA 12 , a very strong GA 12 derivative peak was observed (Fig. 3g ) consistent with the high expression levels observed in this line (Supplementary Fig. 1f ). As a negative control, transient expression of 35 S::GFP in WT protoplasts in the absence of GA 12 did not produce any detectable GA 12 derivative. Quantification of the relative GA 12 derivative peak intensities shows the highest values for the GAS2 -OE1 lines. This is as expected, since strong GAS2 expression is seen in all protoplasts, and the lower values observed in the transient expression experiments using 35 S::GAS2-GFP can be explained by the relatively low efficiency of protoplast transformation (Fig. 3g ). The control experiment, transient expression of GFP in the presence of GA 12 produced very low levels of GA 12 derivative (Fig. 3g ). Fig. 3 Analysis of products produced by the catalytic conversion of GA 12 by GAS2 in vivo and in vitro. a – d LC-MS base peak chromatogram of the products generated by the catalytic conversion of GA 12 by GAS2 at different time intervals (0, 5, 30, and 120 min). [17,17- 2 H 2 ]-GA 12 was used in this assay. e LC-MS dynamic analysis of GA 12 and GA 12 derivative in the reaction solution at different time intervals (0, 5, 30, and 120 min). LC-MS liquid chromatography/mass spectrometry. f – i GA 12 and GA 12 derivative detection using MALDI FTICR-MS spectra in 35 S::GAS2-GFP (GAS2-GFP) ( f ), 35 S::GFP ( i ) transiently transformed in protoplasts and GAS2- OE1 plants ( g ) with GA 12 (2.5 μg/mL), 35 S::GFP transiently transformed into protoplasts was used as a negative control without GA 12 treatment ( h ). j Relative intensity of GA 12 derivative in Arabidopsis protoplasts transiently transformed with 35 S::GAS2-GFP (GAS2-GFP) and 35S::GFP (GFP) overnight. The protoplasts from GAS2 -OE1 plants (GAS2-OE1) were used as a control. GA 12 (2.5 μg/mL) was supplemented as the substrate for GA 12 derivative synthesis catalyzed by GAS2. Values shown are means ± SD ( n = 3). * p < 0.05, t test. Source data are provided as a Source Data file Full size image To further investigate whether GA 12 is an endogenous substrate for GAS2, we transiently expressed a GAS2-GFP fusion protein ( 35 S::GAS2-GFP ) in tobacco ( Nicotiana tabacum ) leaves. Protoplasts isolated from these leaves were incubated in medium containing GA 12 . LC-MS analysis identified appearance of a peak of an m/z 349.20 at a retention time of 2.04 min (Supplementary Fig. 9 ). In contrast, transient expression of 35 S::GFP in tobacco leaves in the presence of GA 12 did not produce any peaks of m/z 349.20 at the 2.04 min retention time (Supplementary Fig. 9 ). Taken together, MALDI FTICR-MS and LC-MS data demonstrate that the presence of the GA 12 derivative is caused by enzymatic conversion of GA 12 by endogenous GAS2 (Fig. 3 and Supplementary Fig. 8 ). In addition, we detected natural occurrence of this GA 12 derivative in maize seedlings proving that GA 12 derivative is present in other plant species (Supplementary Fig. 10 ). Together, our results demonstrate that GAS2 can use GA 12 as substrate for production of an intermediate in GA biosynthesis both in vivo and in vitro. Identification of DHGA 12 structure Purified products from the biosynthetic reactions were analyzed by LC-MS showing a characteristic retention time of 4.85 min (Fig. 4b ). The molecular formula of the GA 12 derivative (GA 12 16,17-dihydro-16α-ol, DHGA 12 ) was inferred to be C 20 H 30 O 5 from the addition of H 2 O to GA 12 resulting in the hydration of the 16, 17-double bond (Fig. 4a–c and Supplementary Fig. 11 ). The existence of GA 12 hydration activity for GAS2 was surprising, and we therefore sought further confirmation of our findings. Analysis of the product from a separate chemical synthesis reaction supported our findings (Fig. 4d–f ). The major product structure of the synthesis reaction according to Markovnikov’s rule should be identical to DHGA 12 (hereafter named DHGA 12C , with the addition of the C subscript to denote chemically synthesized DHGA 12 ) (Fig. 4a, d ), which has been widely reported in previous studies as a classical electrophilic addition reaction [23] , [24] . DHGA 12 and DHGA 12C have identical retention times (Fig. 4b, e ) and TOF MS/MS spectra (Fig. 4c, f ), consistent with identical molecular structures. For further confirmation, we performed NMR assays with the product from chemical synthesis, including 1 H NMR, 13 C NMR, 1 H- 1 H NOESY, 1 H- 1 H COSY, 1 H- 13 C HMQC, and 1 H- 13 C HMBC spectra. From the corresponding 2D NOESY spectrum of DHGA 12 , cross-peaks between the proton H of C-14/C-15 and the proton H of C-17 are not observed, indicating a hydroxyl group on C-16α (Supplementary Figs. 12 – 19 ). DHGA 12 is a C 20 -GA lacking the 4,10-lactone and a hydroxyl group (-OH) at C-3 in the β-orientation characteristic of traditional bioactive GAs (e.g. GA 1 , GA 3 , GA 4 and GA 7 ) (Fig. 4g inset a green oval). Searches in available databases and literature failed to find a compound with a structure and stereochemical configuration identical to DHGA 12 , therefore identifying it as an atypical gibberellin [12] , [25] , [26] . Fig. 4 LC-MS analysis of the new gibberellin, DHGA 12 and its position within the GA biosynthetic pathway. a Schematic of the GAS2-catalyzed conversion of GA 12 to DHGA 12 . Cofactor: 24 µL, containing 133 mM 2-oxoglutarate, 133 mM ascorbate, 16.7 mM FeSO 4 , and 33.3 mg/mL catalase. b Total ion chromatogram (TIC) of DHGA 12 by LC-MS. c MS spectrum of the peak at 4.85 min (retention time) in ( b ). d Schematic of the chemical synthesis of DHGA 12C (subscript C denotes chemically synthesized DHGA 12 ). The chemical synthesis was conducted in the phosphoric acid solution (0.125 mol/L) at 60 o C for 8 h. e TIC of DHGA 12C by LC-MS. f MS spectrum of the peak at 4.85 min (retention time) in ( e ). g The stereochemical configuration of DHGA 12 (green oval) and gibberellin biosynthetic pathway including the GAS2-catalyzed production of DHGA 12 . 20ox GA 20-oxidase, 3ox GA 3-oxidase, 2ox GA 2-oxidase, LC-MS liquid chromatography/mass spectrometry, GA gibberellins, MS Murashige and Skoog agar Full size image In vivo subcellular localization experiments indicate that GAS2 is located in the cytoplasm (Supplementary Fig. 20 ), which is consistent with it acting on a C 20 -GA intermediate [27] , [28] . Our data demonstrate that GAS2 exhibits hydration activity using GA 12 as a substrate to produce DHGA 12 . The proposed pathway for DHGA 12 biosynthesis is illustrated in Fig. 4g . In terms of the general GA biosynthetic and catabolic pathway, DHGA 12 is synthesized from GA 12 in a reaction catalyzed by GAS2 in the cytoplasm, and represents a new branch in the pathway (Fig. 4g ). DHGA 12 is a bioactive GA Since GAS2 can catalyze formation of DHGA 12 from GA 12 (Fig. 4g ), and given the observed phenotypes for gas2 and GAS2- OE, we postulated that DHGA 12 is a bioactive GA, and alterations in DHGA 12 could affect seedling development and ABA responses. To test our hypothesis, we first investigated the effect of exogenous application of DHGA 12 on Arabidopsis cotyledon greening, using seedlings grown in MS medium supplemented with 0 and 0.2 µM ABA (Fig. 5a–d and Supplementary Fig. 21 ). As seen in GAS2 -OE plants, exogenous application of DHGA 12 to WT seedlings stimulates cotyledon greening and counteracts the inhibitory effect of ABA. Furthermore, the delayed cotyledon greening observed in gas2-1 and gas2-2 mutants was partially rescued by the addition of exogenous DHGA 12 . Similar effects were also observed following exogenous application of GA 4 , a GA known to be bioactive (Fig. 5a–d and Supplementary Fig. 21 ). To test whether DHGA 12 is bioactive in hypocotyl elongation, seeds of wild-type, and gas2-1 and gas2-2 mutants, were directly plated on MS, with or without the addition of GA 4 or DHGA 12 , and grown under continuous far-red light (FRL) illumination. Treatment with GA 4 or DHGA 12 significantly promoted hypocotyl elongation in all the tested genotypes (Fig. 5e, f ). Promotion of elongation was less effective in gas2-1 and gas2-2 mutants than in WT plants. In addition, the effects of DHGA 12 on plant growth and ABA response were less pronounced than that of GA 4 . Fig. 5 DHGA 12 antagonistically suppresses the effect of ABA in seedling establishment. a , b Effects of exogenous application of DHGA 12 and GA 4 on cotyledon greening of wild-type, gas2-1 , and gas2-2 , germinated 10-d on MS and MS + 0.2 µM ABA, with or without the addition of DHGA 12 or GA 4 . Bars = 1.5 cm. c , d Cotyledon greening analysis of wild-type, gas2-1 , and gas2-1 , grown on MS at day 4 ( c ) and MS + 0.2 µM ABA at day 7 ( d ), with or without the addition of DHGA 12 or GA 4 . Error bars represent SD ( n = 72, t test, * P < 0.05). Values are the mean of three independent experiments. e , f Effects of exogenous application of DHGA 12 and GA 4 on hypocotyl elongation of 5-d wild-type, gas2-1 and gas2-2 seedlings grown under continuous far-red light illumination. Data represent means ± SD ( n = 22, t test, * P < 0.05). Source data are provided as a Source Data file. ABA abscisic acid Full size image GA 4 , as a bioactive GA, has been shown to bind the GA receptor (GID1) to perform its biological roles [29] . Since DHGA 12 may play a role as a bioactive GA in seedling development, we tested whether it can bind GID1. Firstly, we analyzed the structural similarities between DHGA 12 and two bioactive GAs (GA 3 and GA 4 ) and its precursor GA 12 . Although comparison of the chemical structure of DHGA 12 with those of other bioactive GAs (GA 3 and GA 4 ) demonstrated a different structure (Supplementary Fig. 22a–d ), the DHGA 12 molecule still shared considerable structural similarities. Further in silico analysis of the GID1a-DHGA 12 complex suggested a binding energy of −8.39 kcal/mol, indicating thermodynamic conditions favorable for binding between DHGA 12 and the GA receptor (Supplementary Fig. 22e ). This was confirmed by a direct DHGA 12 to GID1 binding assays using microscale thermophoresis (MST). A functional GID1 homolog, GID1c was purified and tested for its binding to DHGA 12 , GA 4 , and GA 12 (a non-bioactive GA that does not bind the receptor). Our results showed that the glutathione S-transferase (GST)-tagged GID1c binds DHGA 12 and GA 4 with dissociation constants EC 50 = 1.45 ± 0.25 µM and EC 50 = 0.68 ± 0.12 µM (± indicates standard deviation, n = 3), respectively, whereas no binding of GA 12 was detected (Fig. 6a ). Fig. 6 DHGA 12 can directly bind to the GA receptor (GID1c). a Microscale thermophoresis (MST) analysis of DHGA 12 and GA4 binding to GID1c. Dissociation constants of DHGA 12 and GA 4 with GID1c are 1.45 ± 0.25 μM and 0.68 ± 0.12 μM, respectively. Error bars represent SD ( n = 3). b , c Effect of exogenous application of 5 μM DHGA 12 and 5 μM GA 4 on hypocotyl elongation of 10-d wild-type and gid1a-1/1b-1 seedlings grown under continuous far-red light illumination. Data represent means ± SD ( n = 15; t test; * P < 0.05). Bar = 1.5 cm. Source data are provided as a Source Data file. GA gibberellins Full size image To further investigate the biological relationship between DHGA 12 and GID1, we employed a double GA receptor mutant ( gid1a-1/ gid1b-1 ) for genetic analyses. Treatment with exogenous DHGA 12 and GA 4 significantly promoted hypocotyl elongation of wild-type seedlings (Fig. 6b, c ). Hypocotyl elongation was reduced in double gid1a-1/gid1b-1 mutant seedlings demonstrating that GA 4 - and DHGA 12 -stimulated hypocotyl elongation is, at least in part, GID1-dependent (Fig. 6b, c ). In addition, the fact that DHGA 12 -enhanced hypocotyl elongation is only partially inhibited in gid1a-1/1b-1 mutants implies that besides GID1a and GID1b, the effect of DHGA 12 may be mediated by the remaining GID1c homolog. GAS2 alters the ABA/GA ratio during seedling development In order to evaluate the ABA/GA balance in different GAS2 genetic backgrounds, WT, noninduced gas2- D and GAS2- OE1 seeds were collected for quantification of endogenous DHGA 12 , ABA, GA 12 , GA 1 , GA 3 and GA 4 levels using HPLC-MS/MS (Fig. 7a–f and Supplementary Fig. 23 ). DHGA 12 levels were virtually undetectable in noninduced gas2 -D samples, but were clearly detectable in WT and experienced a sharp rise in GAS2- OE1 seeds (imbibed in 4 °C overnight) (Fig. 7a and Supplementary Fig. 23a–c ). In contrast, ABA levels in GAS2- OE1 seeds (imbibed in 4 °C overnight) were ~50% lower than that in the WT, whereas noninduced gas2 -D seeds showed higher levels than that in the WT (Fig. 7b and Supplementary Fig. 23d–f ). Furthermore, we found that expression levels for several genes involved in the ABA synthesis pathway (e.g. NCED 3, ABA1 ) were altered in gas2 -D and gas2 -D plants following induction with E2 (Supplementary Fig. 24a ). Compared with WT, GA 12 levels were enhanced in noninduced gas2- D and reduced in GAS2- OE1 seeds (Fig. 7c and Supplementary Fig. 23g–i ), consistent with our hypothesis that GAS2 metabolizes GA 12 to produce DHGA 12 as a branch of the GA 4 biosynthetic pathway (Fig. 4g ). The GA 3 and GA 4 levels showed a strong reduction in GAS2- OE1 seeds, perhaps reflecting the observed decrease in GA 12 levels, which is consistent with the severe reduction in GA20ox1 expression observed in GAS2 -OE1 plants (Supplementary Fig. 24b ) and/or an increase in the conversion of GA 12 to DHGA 12 . GA 1 levels were not altered in any of the studied genotypes (Fig. 7d–f and Supplementary Fig. 23j–r ). We also used imaging mass spectrometry (IMS) to investigate the possible correlation between the GAS2 expression levels and the endogenous GA and ABA levels (Fig. 7g ). Dry seeds, imbibed seeds (3 days at 4 °C, and germinating seeds (3 days at 4 °C + 2 days at 22 °C) of WT, noninduced gas2 -D, and GAS2 -OE1 lines were analyzed to visualize the endogenous amounts of DHGA 12 , GA 3 , GA 4 and ABA in the tissue. DHGA 12 was not detected in dry seeds of WT, consistent with the lack of GAS2 expression in seeds (Supplementary Figs. 4 , 5 ). Increased DHGA 12 levels were observed in imbibed and germinating GAS2 -OE1 seeds compared with WT, whereas the ABA levels appeared to be reduced in GAS2 -OE1 (Fig. 7g , Supplementary Fig. 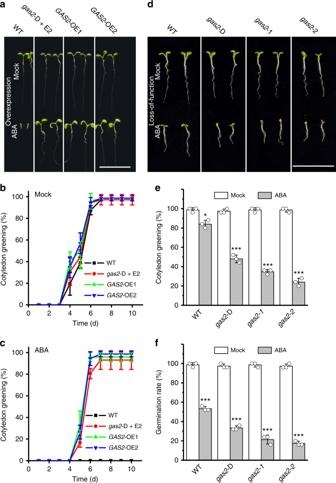Fig. 1 GAS2modulates the sensitivity to ABA in seed germination and seedling establishment.aPhenotypes of 10-d-old seedlings of wild-type, E2-inducedgas2-D and twoGAS2overexpression transgenic lines (GAS2-OE1 and OE2), grown on MS in absence (Mock) or presence of 0.5 µM ABA (ABA). Bar = 1.5 cm.b,cCotyledon greening analysis of 10-d-old seedlings of wild-type, E2-inducedgas2-D and twoGAS2overexpression lines (GAS2-OE1 and OE2) grown on MS with or without the addition of 0.5 µM ABA. Error bars represent SD (standard deviations) (n= 72).dPhenotypes of 8-d-old seedlings of wild-type, noninducedgas2-D,gas2-1andgas2-2, grown on MS in absence (Mock) or presence of 0.2 µM ABA (ABA). Bar = 1.5 cm.eCotyledon greening analysis of 8-d-old seedlings of wild-type, noninducedgas2-D,gas2-1andgas2-2grown on MS in absence (Mock) or presence of 0.2 µM ABA (ABA). Error bars represent SD (standard deviations) (n= 72).fSeed germination analysis of wild-type, noninducedgas2-D,gas2-1andgas2-2, grown on MS in absence (Mock) or presence of 0.2 µM ABA (ABA) at 48 h. Error bars represent SD (standard deviations) (n= 72). E2 stands for 17-β-estradiol. *P< 0.05, ***P< 0.001,ttest versus mock (eandf). Source data are provided as a Source Data file. ABA abscisic acid, MS Murashige and Skoog agar 25 and Supplementary Table 1 ). Taken together, the IMS and HPLC-MS/MS data demonstrated a clear correlation between the ABA/GA ratio upon GAS2 overexpression during dormancy breaking, germination, and early seedling development. Fig. 7 Endogenous GAs and ABA levels in seeds. a – f DHGA 12 , ABA, GA 12 , GA 1 , GA 3 and GA 4 levels in wild-type, noninduced gas2 -D and GAS2 -OE1 seeds. 600 mg Arabidopsis seeds imbibed in 4 °C overnight were used for each sample. Values are expressed as means ± SD (standard deviations) ( n = 3), ** P < 0.01, *** P < 0.001, t test versus WT. g Visualization of ABA, GA 3 , GA 4 and DHGA 12 in wild-type, noninduced gas2 -D and GAS2 -OE1 seeds by MALDI-TOF imaging. Representative images of >3 measurements are presented. Source data are provided as a Source Data file. GA gibberellins, ABA abscisic acid Full size image In this study, we provide a detailed analysis of the interdependence of the effects of ABA and GA on early development using genetic and biochemical approaches, resulting in the identification of GAS2 , a GA-biosynthetic gene, the characterization of its enzymatic activity, the chemical structure of its reaction product, and the establishment of a new route for the biosynthesis of a bioactive intermediate in the GA biosynthesis pathway. The currently accepted paradigm is that the main pathways for the synthesis of bioactive GAs (e.g. GA 1 and GA 4 ) are catalyzed by the GA20ox subfamily [16] , [17] and that the highly biologically active GAs are C 19 -GAs. These all possess a 4,10-lactone, a carboxylic acid (−COOH) at C-6, a hydroxyl group at C-3 in β-orientation, and do not have a hydroxyl group at C-2 in β-orientation. We found that GAS2 uses GA 12 as a substrate to generate a bioactive GA intermediate with a structure different to previously known bioactive GAs. In vitro, GA 12 is converted by GAS2 into a product with a predicted structure that identifies it as a member of the GA family (DHGA 12 ). Unlike most of the known biologically active GAs (GA 1 , GA 3 , GA 4 , and GA 7 ), DHGA 12 is a C 20 -GA, lacking the 4,10-lactone and the β-hydroxyl group (−OH) at C-3 [29] , [30] . Although there are obvious structural differences between DHGA 12 and the known bioactive GAs, we were able to show that DHGA 12 can bind to the GA receptor GID1, albeit with a lower affinity than GA 4 (Fig. 6a ). It has been documented that GID1 receptors evolved from hormone-sensitive lipases through alteration of the substrate-binding pocket to enhance the affinity and specificity for bioactive gibberellins [27] . We have compared our DHGA 12 -GID1a binding simulation results with previous studies [31] , [32] , and found that most of the nonpolar contacts by which GID1a interacts with GA 4 also contact the aliphatic rings of DHGA 12 . Some of the interactions mediated by hydrogen bonds in the GID1a-GA 3 complex, such as Y31, S116, R244, and D245, are also visible in the interaction with DHGA 12 (Supplementary Fig. 22 ). The structural differences between DHGA 12 and other bioactive GAs, such as the lack of the hydroxylated C-3 as well as the lactone ring present in GA 3 and GA 4 , suggest that the molecular interactions between DHGA 12 and receptors have diverged from the established one. The discovery of GAS2 and DHGA 12 highlights the complexity of GA signaling in Arabidopsis , as well as the existence of additional branches in established biosynthetic routes. Further structural research is required to elucidate the details of these interaction mechanisms. Loss-of-function mutations or silencing of GAS2 leads to ABA hyposensitivity while overexpression leads to hypersensitivity (Figs. 1 and 2 ). This is accompanied by a change in the relative amounts of GA and ABA in these lines. Exogenous application of DHGA 12 promotes seed germination, and reverses the FRL-induced inhibition of hypocotyl elongation, albeit to a lesser degree than the bioactive GA 4 . Further work will be needed to determine to what extent these changes are responsible for the observed seedling development phenotypes. These data suggest that DHGA 12 is a bioactive GA or at least a GA that is physiologically relevant. The observations that DHGA 12 is less active as compared to GA 4 , and the partial complementation of the gas2 knockdown lines by exogenous DHGA 12 and GA 4 , imply that there may exist additional factors resulting from the participation of GAS2 in other regulatory processes, perhaps involving interaction with other components of the hormonal metabolism or signaling pathways. It is also possible that additional downstream molecules biosynthesized from DHGA 12 could be the direct cause of our observations. Finally, it cannot be ruled out that GAS2 may have other substrates and products in planta, which possibly contributes to the partial-rescue phenotypes of GAS2 silencing/overexpression lines. Interestingly, the GA-deactivating enzyme CYP714A1 in Arabidopsis [33] and ELONGATED UPPERMOST INTERNODE (EUI) in rice which acts via 16α,17-epoxidation of 13-H GAs [34] could also block the formation of active GAs, such as DHGA 12 , since GAS2 catalyzes GA 12 hydration to DHGA 12 at the 16, 17-double bond. These data imply that GAS2 has function antagonistic to CYP714A1 in Arabidopsis . Conversion of GA 12 to DHGA 12 by GAS2 may therefore represent a GA synthesis/deactivation branch switch for the double bond oxidation. In fact, induction of GAS2 expression led to an increase in DHGA 12 levels and a concomitant reduction in ABA levels while simultaneously decreasing ABA sensitivity, favoring germination over dormancy. This observation points to an important role for GAS2 in the regulation of the balance between the biosynthetic and signaling pathways during germination, with a possible feedback mechanism. Indeed, ABA can induce the expression of GAS2 whereas GA 4 represses GAS2 expression (Supplementary Fig. 5 ). In accordance with the regulatory role discussed above, we noticed a significant decrease in the concentration of the more active GA 4 and ABA in GAS2- overexpressing plants. Firstly, GA 12 is converted to GA 4 through oxidations catalyzed by GA 20-oxidase (GA20ox) and GA 3-oxidase (GA3ox), respectively, whereas we demonstrate that GAS2 also uses GA 12 as a substrate to generate an atypical bioactive DHGA 12 . We speculate that GAS2 and GA20ox1 compete for the available pool of cellular GA 12 . Secondly, hormonal levels undergo dynamic changes in different tissues and development stages. For example, GA 4 concentrations in shoot apices are high in young plants before dropping to very low levels after 2−3 weeks [35] . Shoot apical GA 4 levels also dramatically increase before floral initiation, and continue to rise until reaching ~100 folds increase by day 56. The dynamic changes on GA levels agree with previous data showing that GA 4 is the active GA in the regulation of Arabidopsis shoot growth and floral initiation [11] , [36] , [37] . Similarly, a very substantial decrease in the concentration of the more active GA 4 was found in the seeds of the GAS2 -overexpression line (Fig. 7d–f and Supplementary Fig. 24j–r ). The balance between ABA and GA action serve as the primary determinant of seed dormancy and germination. The relative reduction observed in ABA and GA 4 in the GAS2 -overexpersion plants implies the existence of poorly understood mechanisms controlling the GA/ABA balance. In accordance with this, we found that expression of several ABA synthesis pathway genes (e. g. NCED3 , ABA1 ) was affected in gas2 -D and GAS2 -OE lines. Meanwhile qRT-PCR data indicated that the expression of GA20ox1 was reduced significantly in GAS2 -OE1 plants, consistent with the reduced GA 4 levels observed in GAS2 -OE1 plants (Fig. 7f ). It is well established that active GAs play an important role in the control of seed germination, and the GAS2 overexpression and loss-of-function phenotypes are consistent with the hypothesis that DHGA 12 is the active GA in the regulation of Arabidopsis seedling establishment. Thirdly, the dynamic GA 4 and DHGA 12 could result from distinct hormonal as well as tissue-specific regulation. This study presents genetic and biochemical evidence of the existence of additional, yet undiscovered, bioactive GAs that control plant responses to specific developmental and environmental conditions. One such example is GAS2, catalyzing the synthesis of a bioactive gibberellin (DHGA 12 ). Unlike the structures of traditionally known active GAs, DHGA 12 is a C 20 -GA and lacks the so-called typical 4,10-lactone. Importantly, GAS2-catalyzed hydration of the GA 16, 17-double bond positions this enzyme as a key modulator of the physiological GA/ABA balance, contributing to the control of crucial physiological processes in plants, such as seed dormancy and germination, and the transition from heterotrophic to autotrophic growth. Plant materials and growth conditions Arabidopsis ecotype Columbia (Col-0) was used for this study. The gas2 -D mutant was obtained from an estradiol-inducible activation mutant pool and was isolated by screening seeds on MS medium supplemented with 0.5 μM ABA and 5 μM 17 β-estradiol. The T-DNA insertion site was identified by TAIL-PCR. 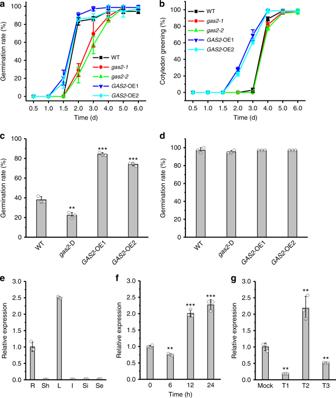Fig. 2 Silencing and overexpression ofGAS2affects seed germination and cotyledon greening.a,bSeed germination and cotyledon greening analysis of wild-type,gas2-1,gas2-2and twoGAS2overexpression lines (GAS2-OE1 and OE2) grown on MS. Error bars represent SD (standard deviations) (n= 72).c,dGermination analysis of wild-type, noninducedgas2-D and overexpressingGAS2fresh seeds (not allowed to dry) at the 2-d timepoint after sowing with no stratification (c) and stratification (at the 3-d timepoint after sowing) (d). Error bars represent SD (n= 108). **p<0.01, ***p<0.001,ttest.eRelativeGAS2mRNA levels in roots (R), shoots (Sh), leaves (L), inflorescences (I), siliques (Si) and seeds (Se) analyzed by RT-qPCR. Error bars represent SD.fRelativeGAS2mRNA levels in hypocotyls ofArabidopsisafter different light/dark treatment (dark 9 d, dark 9 d + light 6 h, dark 9 d + light 12 h and dark 9 d + light 24 h). The dark 9-d level was arbitrarily adjusted to 1 and the remaining levels were normalized to that value. Error bars represent SD. **p< 0.01, ***p< 0.001,ttest.gRelativeGAS2mRNA levels of the seedlings in response to red and far-red light exposure, analyzed by RT-qPCR. Error bars represent SD. **p< 0.01,ttest. Mock: Far red light 0 h; T1: Far red light 2 h; T2: Far red light 2 h + red light 2 h; T3: Far red light 2 h + red light 2 h + Far red light 2 h. Source data are provided as a Source Data file. MS Murashige and Skoog agar Primer sequences are listed in Supplementary Table 2 . For the production of GAS2 overexpression plants, the full-length GAS2 cDNA amplified with the primers of GAS2OE-F and GAS2OE-R was cloned into the binary pBIB vector under the control of the Cauliflower Mosaic Virus 35S promoter. The construct was introduced into Agrobacterium tumefaciens strain GV3101, and Arabidopsis plants transformed using the floral dip method [38] . Primer sequences are listed in Supplementary Table 2 . Unless otherwise specified, seeds used in seed germination tests were sterilized and kept for 3 days at 4 °C in the dark to break dormancy on different media (MS, MS + E2, MS + ABA, MS + ABA + E2) solidified with 0.6% agar. The plates were then transferred to a culture room at 22 ± 2 °C under a 16 h light/8 h dark photoperiod. Seed germination percentages were scored for three independent biological replicates. The hypocotyl length test was performed under far-red light. Seeds were sterilized and kept for 4 days at 4 °C in the dark to break dormancy on the different media (MS, MS + 5 μM DHGA 12 , MS + 5 μM GA 4 ). We employed an LED light source emitting light (FR: 5 μmol/m 2 /s 2 ) with a peak wavelength of 730 nm and a half bandwidth of 25 nm (Quantum Devices). After 5 days, plates were photographed and hypocotyl lengths measured. For the experiments involving measurement of GAS2 mRNA levels in response to red and far-red light exposure. Arabidopsis seedlings were exposed to the following conditions. T1: Far red light 2 h; T2: Far red light 2 h + red light 2 h; T3: Far red light 2 h + red light 2 h + Far red light 2 h. The intensity of the FR light was 60 μmol/m 2 /s 2 , and the intensity of R light was 60 μmol/m 2 /s 2 . Expression levels were determined by RT-qPCR. RNA isolation and expression analyses RNA was isolated from 100 mg tissue samples using the TRIzol reagent (Invitrogen). Total RNA samples (2 μg) were used for reverse transcription with Moloney Murine Leukaemia Virus reverse transcriptase (Promega). Quantitative RT-PCR was used to measure gene transcript levels. Three biological replicates were performed. RT-qPCR was performed using a sequence detector system (7500 Fast, Applied Biosystems) with SYBR Green I. The mean value of three biological replicates was normalized using tubulin as an internal control. The relative quantification method (ΔΔCT) was used to evaluate the relative differences (fold-changes) in transcript levels [39] . Primer sequences are listed in Supplementary Table 2 . GAS2 enzymatic activity and product identification Enzyme assays employed recombinant GAS2 protein, and 10 ng 17-17-[ 2 H 2 ]-labeled GA 12 , 17-17-[ 2 H 2 ]-labeled GA 15 , and 17-17-[ 2 H 2 ]-labeled GA 24 (purchased from Prof. L. Mander, Australian National University, Australia) as substrates, as described previously [40] . In brief, [ 2 H 2 ]GA 12 , [ 2 H 2 ]GA 15 , [ 2 H 2 ]GA 24 was added to the reaction mixtures in the presence of 50 mM Tris, pH 7.8, and a cofactor mixture (24 µL, containing 133 mM 2-oxoglutarate, 133 mM ascorbate, 16.7 mM FeSO 4 , and 33.3 mg/mL catalase) in a total volume of 224 µL. Fresh cofactors were added after 2, 4, 6 and 8 h (24, 24, 24 and 104 µL, respectively). Then the reaction mixtures were incubated at 30 °C overnight and extracted three times. The products were analyzed by liquid chromatography/mass spectrometry (LC-MS) (LCQ Deca AMX, HPLC-electrospray ionization (ESI)–MS, Thermo-Finnigan, USA) [41] . MS-MS data were analyzed using Xcalibur 2.1 software (Thermo-Finnigan). The retention times of samples were compared to deuterium-labeled GA standards. Microscale thermophoresis (MST) Fluorescent labeling was performed using reactive RED dye (NT-647) following the manufacturer’s protocol (Nanotemper, Germany). The labeling procedures were optimized for the GID1c protein to give about 2 tracer molecules per protein, as described by the manufacturer (Nanotemper, Germany). Free dye was removed by Sephadex G-25 column chromatography. MST assays were carried out as described previously [42] , except that serial dilutions of unlabeled GA 4 , GA 12 , and DHGA 12 were respectively mixed with 200 nM of NT-647-labeled proteins in buffers containing 20 mM Tris-HCl (pH 8.0), 200 mM NaCl, and 0.05% Tween-20. MST data were analyzed using the Hill equation. Molecular docking simulations To examine the interaction of GID1a and DHGA 12 , a model of GID1a was obtained from the X-ray crystallographic structure of GID1a [32] , as downloaded from the RCSB Protein Data Bank (2ZSH) at a resolution of 1.80 Å. GA 3 and water molecules were removed from the protein structure for the docking simulations; the protein was regarded as ligand-free. Docking simulations were performed using Autodock 4.2 with AutoDockTools [43] , [44] , [45] . The GID1a grid box was set according to the similar part of the GA 3 binding pocket in the GID1a-GA 3 complex [32] . The number of 20 modes was selected for each docking run. Other parameters were set to their default values. The pose with lowest energy of binding or binding affinity was extracted and the best binding energy was acquired. MALDI-FTICR MS analysis For GA 12 and DHGA 12 detection, cell lysates were extracted from protoplasts transiently transformed with 35 S::GAS2-GFP or 35 S::GFP , and from protoplasts prepared from transgenic plants overexpressing 35 S::GAS2 . The GA 12 substrate (OlChemIm, Czech Republic) was incubated with cell lysate in a total reaction volume of 4 mL, at 22 °C for 16–20 h. The reaction mixture was then broken by addition of 100 μL 90% MeOH, followed by incubation at 4 °C overnight. MALDI-FTICR MS analysis was performed on the supernatant fractions, using a dried-droplet sample preparation protocol: 1 μL of sample solution was mixed with 1 μL of matrix solution, and 1 μL mixture was then pipetted onto the stainless steel target probe, followed by drying under a stream of nitrogen gas at room temperature. A 9.4T Solari X MALDI-FTICR MS (Bruker) equipped with a SmartBeam Nd: YAG 355 nm laser was utilized. The laser was fired at a repetition rate of 2000 Hz. The negative-ion mass spectra in reflectron mode were collected with a pulsed ion extraction time of 200 ns, an accelerating voltage of 19.0 kV, an extraction voltage of 16.6 kV, a lens voltage of 8.0 kV, and a reflector voltage of 21.0 kV. The mass spectra data were acquired over a mass range of m/z 200–600 Da with a resolving power of 1000 Hz (using a 6.71 s time-domain transient length) and visualized using Compass Data Analysis 5.0 (Bruker Daltonics, Billerica, MA) [46] . GA and ABA measurement Six hundred milligrams of dry seeds was used for GA and ABA measurement following previous methods with slight modifications [47] . Six hundred milligrams of dry seeds was imbibed at 4 °C overnight. Samples were then frozen and were ground in liquid nitrogen using a mixer mill MM400 (RetschGmbH, Haan, Germany) in 2 mL Eppendorf tubes. The resultant powder was extracted with 1 mL of extraction solvent (methanol: H 2 O, 90:10 (v/v)) using ultrasonication (4–7 °C). The labeled forms of the compounds d6-ABA, d2-GA 1 , d2-GA 3 , d2-GA 4 , and d2-GA 12 were added as internal standards. After centrifugation (10,000 × g for 15 min at 4 °C), the supernatant was collected, the pellet was re-extracted with 0.5 mL of extraction solvent, and the extraction repeated three times. The supernatants were combined and dried thoroughly under a nitrogen stream, then re-dissolved in 300 μL of methanol before being subjected to centrifugation (10,000 × g for 5 min at 4 °C) and filtration through a 0.22 μm PTFE filter (Waters, Milford, MA, USA). Samples (5 μL) were analyzed using liquid chromatography/mass spectrometry (LCQ Deca AMX, high-performance liquid chromatography (HPLC)-electrospray ionization (ESI)-MS, AB SCIEX-4000 QTRAP, USA). Hormones were measured from two independent samples for each treatment [48] , [49] . Quantification was performed using calibration curves including each of the five unlabeled analytes (ABA, GA 1 , GA 3 , GA 4 , and GA 12 ). 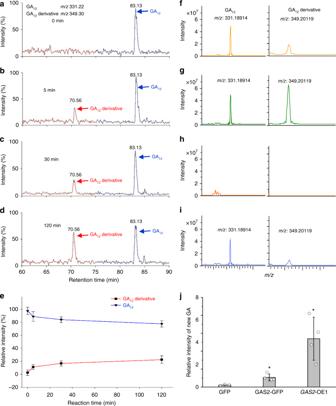Fig. 3 Analysis of products produced by the catalytic conversion of GA12by GAS2 in vivo and in vitro.a–dLC-MS base peak chromatogram of the products generated by the catalytic conversion of GA12by GAS2 at different time intervals (0, 5, 30, and 120 min). [17,17-2H2]-GA12was used in this assay.eLC-MS dynamic analysis of GA12and GA12derivative in the reaction solution at different time intervals (0, 5, 30, and 120 min). LC-MS liquid chromatography/mass spectrometry.f–iGA12and GA12derivative detection using MALDI FTICR-MS spectra in35S::GAS2-GFP(GAS2-GFP) (f),35S::GFP(i) transiently transformed in protoplasts andGAS2-OE1 plants (g) with GA12(2.5 μg/mL),35S::GFPtransiently transformed into protoplasts was used as a negative control without GA12treatment (h).jRelative intensity of GA12derivative inArabidopsisprotoplasts transiently transformed with35S::GAS2-GFP(GAS2-GFP) and 35S::GFP (GFP) overnight. The protoplasts fromGAS2-OE1 plants (GAS2-OE1) were used as a control. GA12(2.5 μg/mL) was supplemented as the substrate for GA12derivative synthesis catalyzed by GAS2. Values shown are means ± SD (n= 3). *p< 0.05,ttest. Source data are provided as a Source Data file Quantitative analysis of GA and ABA by HPLC-MS/MS was performed using 2 H-labeled GAs and d6-ABA as internal standards [38] , [39] . As commercial DHGA 12 is unavailable, DHGA 12 quantification was performed using [ 2 H 2 ] GA 12 as an internal standard. GA and ABA levels were determined in triplicate, independent seed samples, by liquid chromatography tandem mass spectrometry (LC-MS) [50] . Chemical reaction and structure identification GA 12 (4 mg) was dissolved in 4.0 mL methanol by ultrasonication and transferred to a reaction flask. Subsequently, 500 µL H 3 PO 4 (1.0 mol/L) and 3.5 mL water were added to the flask followed by stirring at 700 rpm on a water bath at 60 °C for 8 h. The mixture was separated and detected by LC-MS in negative mode with a full scan from 100 to 500 Da. The structure of DHGA 12C was identified using Waters MassLynx 4.1 software of Waters ACQUITY UPLC H-Class and Waters SYNAPT G2-Si HDMS. MALDI-TOF MS Samples comprising 11 seeds were selected from dry, vernalized, and germinating Arabidopsis seeds; these seed samples were treated as three biological replicates with separate sample preparation and measurement. Measurements were performed using a Time-of-Flight mass spectrometer (Bruker Daltonics, Autoflex Speed) in reflectron mode. The instrument was equipped with a pulsed, 352 nm solid-state laser (Bruker Daltonics, 2 kHz SmartBeam II) operated at a repetition rate of 2000 Hz and a laser pulse energy of 100–190 μJ. The spatial resolution was kept in imaging mode (20 μm), and mass spectra recorded from 500 laser shots for each spot using the default random walk method (Bruker, FlexImaging 4.0). Spectra were recorded in negative-ion mode at 150–400 m/z range. The operating voltage conditions in reflection mode were as follows: ion source 1, 18.95 kV; ion source 2, 16.55 kV; lens, 8.01 kV; reflector 1, 21.02 kV; reflector 2, 9.79 kV. The delay time was 200 ns. Seed samples were individually split into halves using a razor blade. The tissue surface was selected for imaging based on a dry appearance with no bright and visible liquid on its surface. Materials were transferred to an ITO glass slide surface, by allowing the two surfaces to touch each other for 1 s, followed by sample removal and drying of the target by nitrogen flow. All imaging data were normalized with the total ion chromatogram; the highest normalized value of all MS was set to 100%. Matrix solution NEDC ( N -(1-naphthyl) ethylenediamine dihydrochloride), in a 3:7 mixture of ethanol and water, was sprayed over the sample using an ImagePrep automatic matrix sprayer (Bruker) until the entire tissue surface was homogeneously covered. Generation of CRISPR lines The CRISPR construct was designed and produced to generate the knockout mutants [51] . To genotype CRISPR-induced mutations, a 538-bp region including the guide RNA site was amplified by PCR and sequenced by Sanger sequencing. T 2 homozygous mutant plants were obtained and confirmed by sequencing. The sgRNA sequence and genotyping primers for GAS2 are listed in Supplementary Table 2 . Subcellular localization Protoplasts were isolated from Arabidopsis leaves and transformed with a GAS2-GFP fusion constructs [52] . Fluorescence was examined using a laser scanning confocal microscope (LSM710, Zeiss, Germany). The protoplasts were excited at 488 nm and fluorescence was detected at 500–550 nm for GFP. The transmission fields were collected simultaneously for use in merged images. GUS staining Transgenic lines containing the GAS2pro :: GAS2 - GUS constructs were tested for GUS activity by incubation in GUS staining buffer (3 mmol/L 5-bromo-4-chloro-3-indolyl β-glucuronic acid, 0.1 mol/L sodium phosphate buffer, pH 7.0, 0.1% Triton X-100, and 8 mmol/L β-mercaptoethanol) at 37 °C overnight in darkness. Staining was terminated by replacement of the staining solution with 70% ethanol, and the samples were stored at 4 °C until observation under the microscope. Phylogenetic analysis Protein sequences were retrieved from the Arabidopsis protein database and searches for similar sequences was performed by BLAST analysis. Phylogenetic trees were generated using MEGA7 software [53] . Statistical support for the nodes on the Neighbor-Joining trees were evaluated by bootstrap analysis. Protein alignment COBALT software [54] was used to perform multiple alignment of protein sequences using default parameters. The Hidden Markov Model (HMM) profiles of the DIOX_N (PF14226) and 2OG-FeII_Oxy (PF03171) domains were downloaded from the pfam website ( http://pfam.xfam.org/ ). The positions of the DIOX_N and 2OG-FeII_Oxy domains were determined by using HMMSEARCH [55] . DHGA 12 measurement To further investigate whether GA 12 is an endogenous substrate for GAS2, the GAS2-GFP fusion ( 35 S::GAS2-GFP ) and the 35 S::GFP control were respectively infiltrated into tobacco leaves for agrobacterium-mediated transformation. 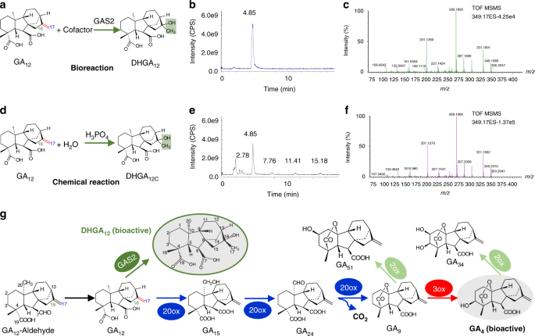Fig. 4 LC-MS analysis of the new gibberellin, DHGA12and its position within the GA biosynthetic pathway.aSchematic of the GAS2-catalyzed conversion of GA12to DHGA12. Cofactor: 24 µL, containing 133 mM 2-oxoglutarate, 133 mM ascorbate, 16.7 mM FeSO4, and 33.3 mg/mL catalase.bTotal ion chromatogram (TIC) of DHGA12by LC-MS.cMS spectrum of the peak at 4.85 min (retention time) in (b).dSchematic of the chemical synthesis of DHGA12C(subscript C denotes chemically synthesized DHGA12). The chemical synthesis was conducted in the phosphoric acid solution (0.125 mol/L) at 60oC for 8 h.eTIC of DHGA12Cby LC-MS.fMS spectrum of the peak at 4.85 min (retention time) in (e).gThe stereochemical configuration of DHGA12(green oval) and gibberellin biosynthetic pathway including the GAS2-catalyzed production of DHGA12. 20ox GA 20-oxidase, 3ox GA 3-oxidase, 2ox GA 2-oxidase, LC-MS liquid chromatography/mass spectrometry, GA gibberellins, MS Murashige and Skoog agar Following infiltration, these transformed tobacco plants were cultured at 22 °C for 16–20 h under continuous light conditions for 3 days [56] and protoplasts were then isolated from the leaves [57] . The detached protoplasts from these samples were treated with 2.5 µg/mL overnight to detect the GA intermediate. The reaction mixture was then broken by addition of 100 μL 90% MeOH. All data were obtained using a Q Exactive™ Hybrid Quadrupole-Orbitrap™ Mass Spectrometer (ThermoFisher) equipped with C18 column (100 cm × 2.1 mm, 1.7 μm), with methanol and water (85/15, v/v) as the mobile phase (0.2 mL/min). NMR The one-dimensional 1 H and 13 C NMR spectra were recorded at 298 K on a Bruker 850 MHz spectrometer equipped with a triple resonance 5 mm HCN-cryoprobe. The chemical shifts were referenced to 0.1% internal tetramethylsilane (TMS). The two-dimensional NMR spectra including NOESY, COSY, HMQC, and HMBC were recorded at 298 K on Bruker 600 MHz spectrometer equipped with a triple resonance 5 mm HCN-cryoprobe. All 2D spectra were collected with 256 × 4096 matrix with 32 or 40 transients per t1 increment. 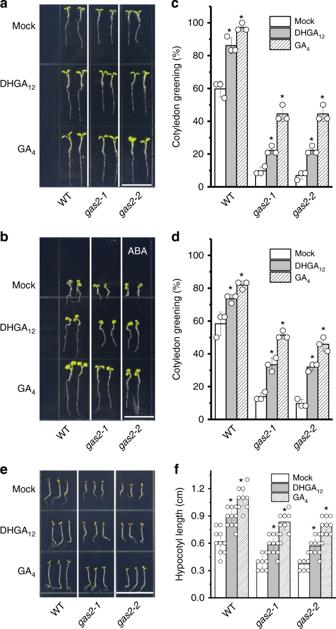Fig. 5 DHGA12antagonistically suppresses the effect of ABA in seedling establishment.a,bEffects of exogenous application of DHGA12and GA4on cotyledon greening of wild-type,gas2-1, andgas2-2, germinated 10-d on MS and MS + 0.2 µM ABA, with or without the addition of DHGA12or GA4. Bars = 1.5 cm.c,dCotyledon greening analysis of wild-type,gas2-1, andgas2-1, grown on MS at day 4 (c) and MS + 0.2 µM ABA at day 7 (d), with or without the addition of DHGA12or GA4. Error bars represent SD (n= 72,ttest, *P< 0.05). Values are the mean of three independent experiments.e,fEffects of exogenous application of DHGA12and GA4on hypocotyl elongation of 5-d wild-type,gas2-1andgas2-2seedlings grown under continuous far-red light illumination. Data represent means ± SD (n= 22,ttest, *P< 0.05). Source data are provided as a Source Data file. ABA abscisic acid 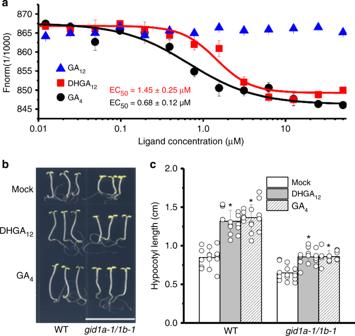Fig. 6 DHGA12can directly bind to the GA receptor (GID1c).aMicroscale thermophoresis (MST) analysis of DHGA12and GA4 binding to GID1c. Dissociation constants of DHGA12and GA4with GID1c are 1.45 ± 0.25 μM and 0.68 ± 0.12 μM, respectively. Error bars represent SD (n= 3).b,cEffect of exogenous application of 5 μM DHGA12and 5 μM GA4on hypocotyl elongation of 10-d wild-type andgid1a-1/1b-1seedlings grown under continuous far-red light illumination. Data represent means ± SD (n= 15;ttest; *P< 0.05). Bar = 1.5 cm. Source data are provided as a Source Data file. GA gibberellins 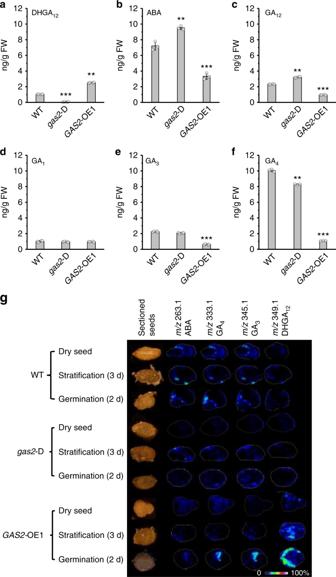Fig. 7 Endogenous GAs and ABA levels in seeds.a–fDHGA12, ABA, GA12, GA1, GA3and GA4levels in wild-type, noninducedgas2-D andGAS2-OE1 seeds. 600 mgArabidopsisseeds imbibed in 4 °C overnight were used for each sample. Values are expressed as means ± SD (standard deviations) (n= 3), **P< 0.01, ***P< 0.001,ttest versus WT.gVisualization of ABA, GA3, GA4and DHGA12in wild-type, noninducedgas2-D andGAS2-OE1 seeds by MALDI-TOF imaging. Representative images of >3 measurements are presented. Source data are provided as a Source Data file. GA gibberellins, ABA abscisic acid NOESY spectra were acquired using mixing times of 1 s. The long-range coupling value for HMBC spectra was set to 8 Hz. Reporting summary Further information on experimental design is available in the Nature Research Reporting Summary linked to this article.